Twin-induced one-dimensional homojunctions yield high quantum efficiency for solar hydrogen generation Efficient charge separation is of crucial importance for the improvement of photocatalytic activity for solar hydrogen evolution. Here we report efficient photo-generated charge separation by twin-induced one-dimensional homojunctions with type-II staggered band alignment, using a ternary chalcogenate, i.e. Cd 0.5 Zn 0.5 S nanorod as a model material. The quantum efficiency of solar hydrogen evolution over this photocatalyst, without noble metal loading, reaches 62%. Unlike traditional heterojunctions, doping or combination of additional elements are not needed for the formation of this junction, which permits us to tune the band structures of semiconductors to the specific application in a more precise way. Our results highlight the power of forming long-range ordered homojunctions at the nanoscale for photocatalytic and photoelectrochemical applications. As Fujishima and Honda [1] first presented the concept of photo-electrochemical water splitting into H 2 and O 2 over a TiO 2 electrode, photocatalytic hydrogen production from water by semiconductors has attracted considerable interest [1] , [2] , [3] , [4] , [5] , [6] . To date, a number of semiconductor photocatalysts including sulfides, nitrides, metal/metallic oxides, and others have been investigated [1] , [7] , [8] , [9] , [10] , [11] , [12] , [13] , [14] , [15] . However, further commercial development, as well as large scale manufacture of photocatalysts, is still restricted by their low activity and high cost. Photocatalytic reaction over semiconductors is usually considered as the direct absorption of a photon by the energy band gap of materials. Upon photon excitation, the separated electron and hole migrate to the semiconductor surface where photocatalytic reactions occur [6] . Therefore, at the most basic level, enhancing charge separation and preventing their recombination before they move to the surface-reactive sites of the photocatalyst have key roles in determining the solar energy conversion efficiency. To this end, many strategies have been investigated, including in situ photodeposition of noble metal as cocatalysts onto photocatalyst surface, chemical doping to form donor or acceptor energy levels within the band gap of the photocatalyst, and development of Z-scheme systems [16] , [17] , [18] , [19] , [20] . Among these approaches, coupling of two different materials or phases at the nanoscale to form heterojunctions has proven successful, owing to improved interfacial charge transfer and therefore effective charge separation [20] , [21] , [22] , [23] . However, because of the random and disordered distributions of heterojunctions within these materials, it could be speculative to solely attribute the observed difference in photocatalytic activity to the existence of the junctions. On the other hand, doping or combination of additional elements is often needed for the formation of these hetero-junctions, making it difficult to precisely tailor the band structures of semiconductors to the specific application. Twinning in nanocrystals, especially in one-dimensional (1D) nanomaterials, has been investigated over III–V and II–VI semiconductors anticipating their potential applications in optical and electronic devices [24] , [25] , [26] . Usually, twin planes periodically occur with a constant spacing and have a long-range order, resulting in twinning superlattice (TSL) in a specific dimension [24] , [25] , [26] , [27] , [28] , [29] . Thus, mini-bands could be generated in this crystal structure [24] . Calculation also reveals that unusual states of charge carriers may emerge from the twinning plane as electron wavefunction is discontinuous around this domain [30] . 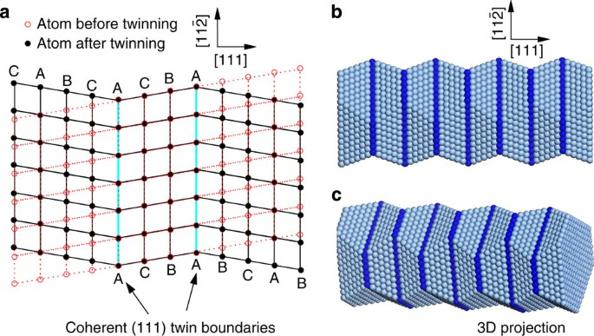Figure 1: Structural models of a typical twin nanocrystal. (a) Two (111)/[11-2] type coherent twin planes involved in a zinc blende (ZB) FCC lattice matrix. The thicker cyan lines represent twin planes. Red circles and solid black solid are lattice configurations before and after twining, respectively. Structurally, twin planes within one crystal are usually parallel to each other as they index to the same crystal plane. Besides, lattices on one side are symmetrical with that of the other side of the twin plane (like a mirror). (b) A twinned nanorod as seen from the [−110] direction. (c) Three-dimensional projection as observed from a high-index [−hhk] direction. The dark blue layers inb,cindicate the twin planes. Figure 1 presents typical face-centered cubic lattice symmetry with two coherent twin planes parallel to each other (see Fig. 1a ) and the resulting TSL domain in a 1D ‘nanorod’ as viewed from [−110] and high-index [−hhk] directions (see Fig. 1b,c ). Although a convincing example is still needed, we assume that the mini-bands formed by TSL could be very useful for charge separation in photocatalysts. Recently, we found that spherical twin-containing Cd 0.5 Zn 0.5 S photocatalyst without loading noble metal exhibited excellent photocatalytic activity for H 2 evolution, with a quantum efficiency (QE) of 43% at 425 nm (ref. 31 ). Nevertheless, tangible proof for the contribution of nano-twins to charge separation in photocatalytic materials is still highly desired. Moreover, the low density of twin planes and the poorly controlled crystal shape in these twin-containing Cd 0.5 Zn 0.5 S photocatalyts indicate a large space for the further improvement of its photocatalytic efficiency. Figure 1: Structural models of a typical twin nanocrystal. ( a ) Two (111)/[11-2] type coherent twin planes involved in a zinc blende (ZB) FCC lattice matrix. The thicker cyan lines represent twin planes. Red circles and solid black solid are lattice configurations before and after twining, respectively. Structurally, twin planes within one crystal are usually parallel to each other as they index to the same crystal plane. Besides, lattices on one side are symmetrical with that of the other side of the twin plane (like a mirror). ( b ) A twinned nanorod as seen from the [−110] direction. ( c ) Three-dimensional projection as observed from a high-index [−hhk] direction. The dark blue layers in b , c indicate the twin planes. Full size image Here we report a twinned Cd 0.5 Zn 0.5 S anisotropic nanocrystal with controllable aspect ratios and a high proportion of long-range ordered twin planes, which give rise to the alternating zinc-blende (ZB) and wurtzite (WZ) segments along <111> direction of the designed material. Further investigations reveal that the type-II staggered band alignment formed between the ZB and WZ segments, leads to the generation of myriad homojunctions in a specific dimension. These homojunctions were found to be highly efficient in charge separation and photocatalytic hydrogen production with a remarkable QE of 62%. We believe that our findings could also be extended to other semiconductor materials and provide a new and generalized approach for the development of novel active photocatalytic materials. 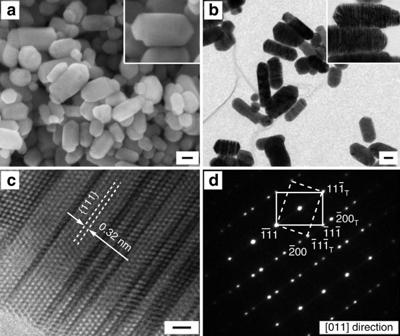Figure 2: Morphology and structure of Cd0.5Zn0.5S nanorod. (a,b) SEM and TEM images of the as-prepared Cd0.5Zn0.5S nanorods with high density of twin planes. (c) HRTEM of the nanorod with {111} twin plane. (d) the selected area electron diffraction (SAED) patterns confirming the formation of (111)/[11-2]-type slips in nano-twins. The insets ina,bare single particles with higher resolution. Scale bars in (a–c) are 50 nm, 50 nm and 1 nm, respectively. Characterizations of twinned Cd 0.5 Zn 0.5 S nanorods Figure 2 shows typical electron microscopic images, as well as selected area electron diffraction patterns, of the Cd 0.5 Zn 0.5 S-EN10 nanocrystals. The scanning electron microscopy (SEM) images ( Fig. 2a ) clearly show the existence of mono-dispersed short nanocrystals in a polygonal cross profile with average diameter of around 60 nm and aspect ratio of 4 (as statistically estimated in Supplementary Fig. S1 ). A closer examination (inset of Fig. 2a ) indicates that the two tips of the nanocrystal were notably different, with the cross-section of one head smaller than that of the main body, and the other gradually tapered to its ends. The anisotropic geometry was also verified by transmission electron microscope (TEM) analysis as shown in Fig. 2b . For simplicity, these anisotropic Cd 0.5 Zn 0.5 S nanocrystals were collectively called ‘nanorods’. The TEM images (inset of Fig. 2b ) further revealed that the ‘nanorods’ consisted of a high density of stacking faults with parallel distribution. The high-resolution TEM image ( Fig. 2c ) showed that most of these parallel dislocations were coherent twin boundaries. The fringes with a lattice spacing of ca. 0.32 nm could be indexed to the {111} planes of the ZB lattice. Further investigation on morphology ( Fig. 2c ) showed that their surfaces were not as smooth as those found in the SEM images. Instead, the nanorods were composed of non-uniformed zigzag structures originating from the suddenly interrupted lattice continuity by twin boundaries. Most of the zigzag segments had a longitude size (spacing) <10 nm due to the high density of twin boundaries (see Supplementary Fig. S2 ). The nano-twin structure was also supported by the selected area electron diffraction pattern shown in Fig. 2d . Ordered spots appeared at the sites one-third from the normal spots known as the diffraction of coherent twins [32] , [33] . Schematic illustration of the crystal structure for this twinned Cd 0.5 Zn 0.5 S nanocrystal obtained by using atomic models is presented in Supplementary Fig. S3 . Clearly, Cd/Zn layers and S layers symmetrically distribute around the twin plane (either the metal layer or S layer) at the center region of the lattice as shown in Supplementary Fig. S3a . Particularly, the deviated atoms after twinning from the original sites should be responsible for the unique diffraction features. Figure 2: Morphology and structure of Cd 0.5 Zn 0.5 S nanorod. ( a , b ) SEM and TEM images of the as-prepared Cd 0.5 Zn 0.5 S nanorods with high density of twin planes. ( c ) HRTEM of the nanorod with {111} twin plane. ( d ) the selected area electron diffraction (SAED) patterns confirming the formation of (111)/[11-2]-type slips in nano-twins. The insets in a , b are single particles with higher resolution. Scale bars in ( a – c ) are 50 nm, 50 nm and 1 nm, respectively. Full size image To confirm the solid solution formation and exclude the possibility of phase segregation between CdS and ZnS, we have carried out the elemental analysis with scanning TEM (STEM) and energy dispersive X-ray (EDX) analysis. According to the mapping and ‘longitude’ and ‘latitude’ line scans over a typical twinning Cd 0.5 Zn 0.5 S nanorod, as shown in Supplementary Fig. S4 , Cd, Zn and S are homogeneously distributed in the Cd 0.5 Zn 0.5 S nanorod, respectively. In addition, the successive shifts of powder X-ray diffraction peaks, as well as ultraviolet-vis absorption edges for other Cd 1- x Zn x S (0≤ x ≤1) nanocrystals, as shown by Supplementary Fig. S5 , provided further proofs of the formation of Cd 0.5 Zn 0.5 S solid solution. Photocatalytic tests over these Cd 1- x Zn x S nanocrystals demonstrated significant improvement in the energy conversion efficiency over Cd 0.5 Zn 0.5 S-EN10 photocatalyst ( Fig. 3a ). The initial hydrogen production rate under visible light irradiation reached 2.58 mmol h −1 with a QE of 62% at 425 nm, as also evidenced by Supplementary Movie 1 . To the best of our knowledge, this is one of the highest efficiency achieved over powdered photocatalysts for visible-light-driven hydrogen production, without employing any cocatalysts. The photocatalyst also have relatively good stability with maintained activity after 25 h of testing ( Fig. 3b ). For those Cd 1- x Zn x S with x <0.5, owing to their lower conduction band (CB) position, less overpotential are available for hydrogen production. On the other hand, x larger than 0.5 are also not favoured due to reduced visible light absorption. Up to now, higher efficiencies have only been reported over Pt/PdS/CdS and PdS/CdS photocatalysts, However, both of them are noble-metal containing [20] . Based on the H 2 generation results in Fig. 3b , we also evaluated the kinetics of the reaction. The rate constant ( k ) was obtained by plotting −ln( C t,Na 2 , S / C 0,Na 2 , S ) against the reaction time, assuming that the reaction fits the first order kinetics and considering that one mole of H 2 generation always corresponds to one mole of Na 2 S consumption [34] . As shown in Supplementary Fig. S6 , the reaction well fitted the first order kinetics with the almost unchanged k values of 0.043 h −1 , 0.038 h −1 , 0.036 h −1 and 0.037 h −1 , respectively, for each run. This again demonstrated the stable photocatalytic behavior of our material. 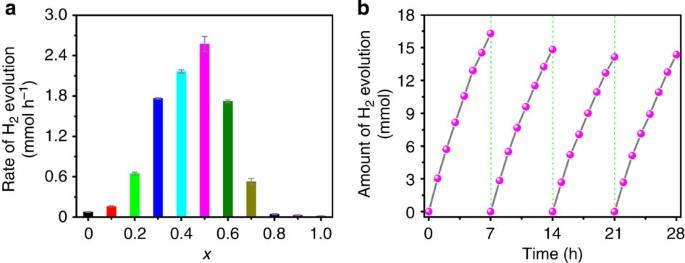Figure 3: Photocatalytic performances of Cd1-xZnxS-EN10. (a) The initial hydrogen generation rate over Cd1-xZnxS solid solutions of various Cd/Zn molar ratios by 5 h test. (b) Time course for hydrogen generation over Cd0.5Zn0.5S-EN10 nanorods. Error bars inaare s.e. values of three tests (n=3). Figure 3: Photocatalytic performances of Cd 1- x Zn x S-EN10. ( a ) The initial hydrogen generation rate over Cd 1- x Zn x S solid solutions of various Cd/Zn molar ratios by 5 h test. ( b ) Time course for hydrogen generation over Cd 0.5 Zn 0.5 S-EN10 nanorods. Error bars in a are s.e. values of three tests ( n =3). Full size image A QE of 43% over spherical Cd 0.5 Zn 0.5 S photocatalyst possessing twinning domain has been reported [31] . Given the isotropic properties of this spherical Cd 0.5 Zn 0.5 S photocatalyst, the formation of TSL with a long-range order is not possible. However, this may be available in 1D material such as nanorods and nanowires. As expected, the high activity of present Cd 0.5 Zn 0.5 S nanorods indicates the significant contribution of long-range TSL-induced charge mobility to the enhanced activity of the photocatalyst. Charge separation over the twin-induced homojunction To understand the relationship between the twinning nanostructures and their resultant performances, the fundamental lattice symmetry of the twin plane in a nanocrystal must be emphasized. In general, binary compounds with close-packed crystal structures can crystallize into ZB, WZ, or their mixtures, in which one layer can be defined as a bilayer composed of paired atoms of its components. For instance, in ZB ZnS, the paired atoms are composed of one Zn atom and one S atom. The lattice sequences of ZB and WZ structures are AaBbCcAaBbCc and AaBbAaBb, respectively (the paired letters, for example, Aa or Bb, represents a bilayer). However, the ordered structures can be broken when stacking faults are introduced. As a twin plane in ZB structure in the <111> direction can be considered as a monolayer of WZ structure [25] , it means that a stacking fault in ZB (WZ) can create a segment of WZ (ZB). For example, in the ZB structure, misplacement of a bilayer to yield a sequence of AaBb Cc Aa Cc BbAc results in a symmetry structure with a mirror plan Aa , which is known as a twin plane or twin boundary, whereas the consequent Cc Aa Cc segment can be recognized as a three-bilayer WZ structure [28] , [35] . Therefore, the appearance of these twin boundaries in nanocrystals can suddenly break the continuity of the ZB lattice constitution and generate a myriad of WZ segments in the ZB lattice. Accordingly, the density of twin planes in these nanocrystals could influence the ratio of WZ/ZB phases. Series of modeling on Cd 1− x Zn x S twinning nanocrystals were thus carried out. The calculations were firstly executed on the twin planes in pure CdS and ZnS nanocrystals, respectively. Linear transformation of band structures from CdS to ZnS was then applied considering the solid solution properties of Cd 1− x Zn x S (0≤ x ≤1). Band structure calculations indicated type-II staggered band alignment around the twin plane, with a CB offset of 46 meV and a valence band offset of 115 meV for CdS, as well as a CB offset of 98 meV and a valence band offset of 39 meV for ZnS. The calculation suggested that WZ Cd 1− x Zn x S could occupy a higher CB and valence band (VB) position than its ZB counterpart. The results were further confirmed by calculations of the plane-averaged charge distribution of the VB maximum (VBM) and CB minimum (CBM) states. As shown in Fig. 4 , the VBM state was more localized in the WZ region (near twin boundary), whereas CBM was more localized in the ZB region (away from twin boundary). These results are in well agreement with those reported for bulk ZnS and CdS semiconductors [36] , [37] . By linear approximation, similar type-II staggered band alignment was obtained in Cd 0.5 Zn 0.5 S, with a WZ CB 106.5 meV above that of ZB and a WZ VB 42.5 meV above that of ZB. The average band gap of the twinning Cd 0.5 Zn 0.5 S nanorod was determined to be 2.62 eV according to the Kubelka-Munk method from the ultraviolet-vis spectrum shown in Supplementary Fig. S5b [38] . 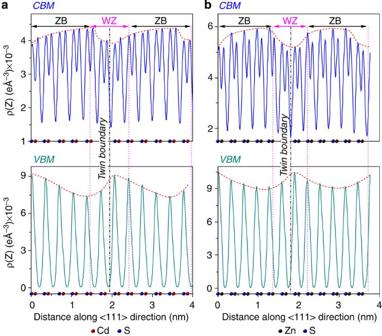Figure 4: Plane averaged charge densities round twin planes. (a) CB minimum (CBM) (up) and VB maximum (VBM) (down) states of zinc blende (ZB) CdS with one twin plane at the center region. (b) CBM (up) and VBM (down) states of ZB ZnS with one twin plane at the center region. Figure 4: Plane averaged charge densities round twin planes. ( a ) CB minimum (CBM) (up) and VB maximum (VBM) (down) states of zinc blende (ZB) CdS with one twin plane at the center region. ( b ) CBM (up) and VBM (down) states of ZB ZnS with one twin plane at the center region. Full size image Based on above analysis, Fig. 5 gives the structural configuration ( Fig. 5a ) and band positions ( Fig. 5b ) for our twinning Cd 0.5 Zn 0.5 S. For comparison, ZB/WZ segments distribution in a real Cd 0.5 Zn 0.5 S nanorod twinning crystals was also provided. As shown by Fig. 5c , periodic light/dark contrast results from alternating twins along the <111> crystalline direction of Cd 0.5 Zn 0.5 S nanorod could be clearly observed. Unlike traditional heterojunctions formed by coupling two different semiconductor materials, the staggered band alignment in our Cd 0.5 Zn 0.5 S was considered to act as a special homojunction, as highlighted in pink regions of Fig. 5 . As illustrated in Fig. 5b , the up-shift of both CB and valence band energy levels for WZ segment compared with that of ZB segments could simultaneously lead to efficient separation of both photo-excited electrons and holes. This is obviously different from most of heterogeneous junctions that can only separate either electrons or holes alone [23] . Large distribution and the close interconnection at the atomic level of two phases (ZB and WZ) and the formation of such homojunctions are believed to favour the vectorial transfer of photo-induced charges, which has been extensively explored by heterojunction design [23] , [26] , [28] , [39] . 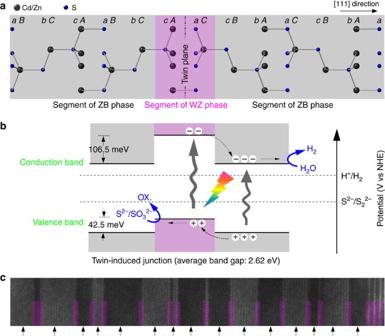Figure 5: Schematics of the homojunction. (a) Ball-stick structure of a typical twin boundary in a zinc blende (ZB) nanorystal to form ZB–WZ–ZB homojunction. (b) Mechanism for photo-generated charge separation over the ZB–WZ–ZB homojunction with staggered band alignment in Cd0.5Zn0.5S photocatalyst. (c) A schematic illustration of the parallel homojunctions in a real Cd0.5Zn0.5S nanorod (from TEM image), the black arrows and pink squares indicate the segments of ZB and WZ structures, respectively. Figure 5: Schematics of the homojunction. ( a ) Ball-stick structure of a typical twin boundary in a zinc blende (ZB) nanorystal to form ZB–WZ–ZB homojunction. ( b ) Mechanism for photo-generated charge separation over the ZB–WZ–ZB homojunction with staggered band alignment in Cd 0.5 Zn 0.5 S photocatalyst. ( c ) A schematic illustration of the parallel homojunctions in a real Cd 0.5 Zn 0.5 S nanorod (from TEM image), the black arrows and pink squares indicate the segments of ZB and WZ structures, respectively. Full size image Formation mechanism of 1D homojunctions Johansson et al . [40] found that higher growth temperatures increased the likelihood of twin formation and in the mass-transport limited process. It is therefore considered that if hydrothermal method is to be used, relatively high hydrothermal treatment temperature is needed. This is the reason why we have chosen hydrothermal treatment temperature of as high as 230 °C. To further investigating the underlying mechanism for the formation of homojunctions in our Cd 0.5 Zn 0.5 S nanorod, we then prepared Cd 0.5 Zn 0.5 S nanocrystals with similar sizes, crystal structures and light absorption properties by simply changing the coordination agent for comparison ( Supplementary Fig. S7 ). For example, twin-plane-free ZB Cd 0.5 Zn 0.5 S nanocrystals with spherical polyhedral shapes (denoted as Cd 0.5 Zn 0.5 S-EN0) and ZB Cd 0.5 Zn 0.5 S twinning nanorods with an aspect ratio of ca. 1.9 (denoted as Cd 0.5 Zn 0.5 S-EN5) were obtained by adding 0 and 5 ml ethylenediamine (EN), respectively. By contrast, twinning ZB Cd 0.5 Zn 0.5 S nanocrystals with spherical polyhedral shapes were obtained by adding NaOH instead of EN (denoted as Cd 0.5 Zn 0.5 S-NaOH; this material has been previously prepared by us using a traditional hydrothermal method [31] ). Clearly, twinning structure cannot be obtained in hydrothermal reaction at 230 °C in the absence of OH − or EN. It indicates that high temperature alone is not enough for the formation of twinning structure and the existence of OH − or EN is also indispensible in the hydrothermal preparation of twinning Cd 0.5 Zn 0.5 S. It has been reported that the difference in mass transportation for the various elements is crucial for the formation of twinning structures. Taking VLS growth of twinning GaP (gold as seed/catalyst) as an example, due to its extremely low solubility in gold, phosphorous has to migrate to the growth interface from the vapor phase to complete the GaP growth. In contrast, Ga has a quite good solubility in gold. Therefore, the growth can be greatly slowed down by the slow mass transportation of P. In this mass-transport limited process, any fluctuations, such as thermal fluctuations could lead to twin-plane nucleation, due to the low energy for the formation of coherent twin plane [40] . In our case, OH − or EN as coordinating agent for Cd 2+ and Zn 2+ ions is also believed to have similar roles. The microwave method employed may lead to more thermal fluctuations in the entire synthesis process and contribute further to the twin plane formation. Moreover, twin planes in the nanocrystal, especially in a nanowire, have been reported to be beneficial for the releasing of the stored elastic energy [26] . These could be additional benefits facilitating the spherical to nanorod morphology transition for our Cd 0.5 Zn 0.5 S nanotwins. It is also noteworthy that EN has played a crucial role for in the formation our 1D-nanorod structure. In fact, similar role of EN has also been found for the formation of many anisotropic structures on various materials, such as nanowire, nanorod, and nanosheet/plate and so on [41] , [42] , [43] , [44] , [45] . It was proposed that atoms on coherent {111} twin plane possessed high coordination number and had relatively low formation energy even comparable to the normal {111} facets [27] , [46] , [47] , [48] . The [111] preferential growth of our twinning Cd 0.5 Zn 0.5 S nanorod is therefore believed to be also due to the capping effect of EN. Comparative validation on the role of 1D homojunctions Photocatalytic tests over these various Cd 0.5 Zn 0.5 S samples were then carried out to evaluate their photocatalytic performances. As shown in Fig. 6a , samples Cd 0.5 Zn 0.5 S-NaOH, Cd 0.5 Zn 0.5 S-EN5 and Cd 0.5 Zn 0.5 S-EN10 exhibited much higher activity than that without twinning structure. This again demonstrated the crucial role of twin-induced junctions in enhancing photocatalytic activity. QEs at 425 nm for the four Cd 0.5 Zn 0.5 S photocatalysts were then evaluated and plotted against the aspect ratio of the various prepared Cd 0.5 Zn 0.5 S nanocrystals. As shown in Fig. 6b , with similar morphology and size, the QE of twinning Cd 0.5 Zn 0.5 S spherical polyhedrons ( ca. 40%) were found to be about 4.4 times that without nano-twins ( ca. 9%). The efficiency can be further improved to 55% over the twinning nanorods with an aspect ratio of 1.9. The highest QE of 62% as aforementioned was obtained over nanorods with an aspect ratio of ~4.0. It is noteworthy that the highest QE reported so far for photocatalytic hydrogen production without noble metal loading is 51% (ref. 16 ). While our photocatalyst reaches 62%. Clearly, the enhanced charge separation and consequent high activity has a close relationship with the large aspect ratios of the twinning nanocrystal. 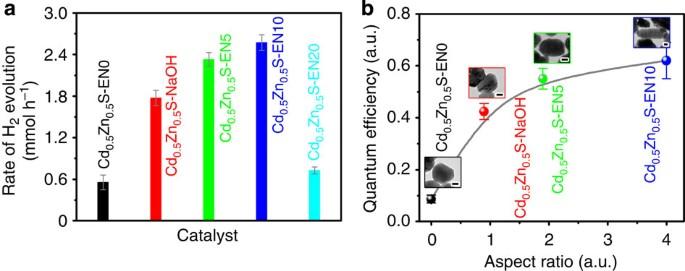Figure 6: Photocatalytic activity of various Cd0.5Zn0.5S samples. (a) The initial hydrogen generation rate of H2evolution over Cd0.5Zn0.5S-EN0, Cd0.5Zn0.5S-NaOH, Cd0.5Zn0.5S-EN5, Cd0.5Zn0.5S-EN10 and Cd0.5Zn0.5S-EN20 with 5 h tests. (b) QEs obtained over Cd0.5Zn0.5S nanocrystals of twin-free spherical polyhedrons, twinning spherical polyhedrons, twinning nanorods with aspect ratio of ca. 1.9, and twinning nanorods with aspect ratio of ca. 4.0, respectively; Calculated QEs are plotted against the average aspect ratios of various Cd0.5Zn0.5S nanocrystals. For the twin-free spherical Cd0.5Zn0.5S nanocrystals, the aspect ratio was defined as zero. Error bars are s.e. values of three tests (n=3). Scale bars for the TEM images in the sets ofbis 20 nm. Figure 6: Photocatalytic activity of various Cd 0.5 Zn 0.5 S samples. ( a ) The initial hydrogen generation rate of H 2 evolution over Cd 0.5 Zn 0.5 S-EN0, Cd 0.5 Zn 0.5 S-NaOH, Cd 0.5 Zn 0.5 S-EN5, Cd 0.5 Zn 0.5 S-EN10 and Cd 0.5 Zn 0.5 S-EN20 with 5 h tests. ( b ) QEs obtained over Cd 0.5 Zn 0.5 S nanocrystals of twin-free spherical polyhedrons, twinning spherical polyhedrons, twinning nanorods with aspect ratio of ca. 1.9, and twinning nanorods with aspect ratio of ca. 4.0, respectively; Calculated QEs are plotted against the average aspect ratios of various Cd 0.5 Zn 0.5 S nanocrystals. For the twin-free spherical Cd 0.5 Zn 0.5 S nanocrystals, the aspect ratio was defined as zero. Error bars are s.e. values of three tests ( n =3). Scale bars for the TEM images in the sets of b is 20 nm. Full size image Time-resolved photoluminescence emission decay spectra, which have been widely used to evaluate the lifetime of photogenerated carriers in semiconducting materials, were then recorded for various Cd 0.5 Zn 0.5 S samples. All the samples were excited at 305 nm and the data were collected at 495 nm, which corresponds to the emission peak of Cd 0.5 Zn 0.5 S. The lifetime ( τ ) was calculated by an exponential decay approach according to the equation I = I 0 e − t / τ + b , where I is the impulse function decay at time t . As shown in Supplementary Fig. S8 , the excited carrier in Cd 0.5 Zn 0.5 S-EN0 presented the shortest lifetime ( τ =2.36±0.12 ns). By contrast, the emission decay times for those Cd 0.5 Zn 0.5 S samples with nano-twins were obviously slowed down. τ is 3.25±0.12 ns for spherical nano-twins and it is 4.02±0.25 ns and 5.41±0.41 ns for twinning Cd 0.5 Zn 0.5 S with aspect ratios of ca. 1.9 and ca. 4.0, respectively. Obviously, twinning nanocrystals with larger aspect ratios will lead to prolonged lifetime of photogenerated charges. More importantly, by plotting QEs as a function of the aspect ratio of TSL in these Cd 0.5 Zn 0.5 S nanocrystals and taking the aspect ratio of non-twin polyhedral Cd 0.5 Zn 0.5 S-EN0 as zero (spherical Cd 0.5 Zn 0.5 S without twin planes), a well-defined upward curve was generated. Figure 6b indicates that a higher aspect ratio of twin photocatalyst, such as nanowire, is expected to result in further improved efficiency. This finding again demonstrated the importance of long-range ordered TSL for the enhancement of photocatalytic activity, which cannot be obtained in traditional spherical structures as we have previously reported for twinning Cd 0.5 Zn 0.5 S nanoparticles [31] . The activity of photocatalytic process has long relied on the crystal structure of semiconductors to facilitate charge separation. As aforementioned, the unique twin induced TSL with a long-range order has been obtained by our EN-assisted high-temperature hydrothermal preparation. The resultant homojunctions could lead to significantly enhanced photocatalytic activity. Both our theoretical and experimental investigations have provided direct proof of the crucial role of twin-induced homojunction in prompting charge separation and photocatalytic reactions. As shown in Fig. 5b , the photogenerated electrons and holes can be spatially separated to the ZB (away from the twin plane) and WZ (to twin plane) regions, respectively, because of the presence of this homojunction. On the other hand, semiconductors with one dimensional (1D) nanostructures (corresponding large aspect ratios) have been proposed to have higher charge-separation ability than their bulk counterpart [49] , [50] , [51] . For our Cd 0.5 Zn 0.5 S twinning nanorods, ordered long-range twinning planes with preferred orientation of [111] direction were achieved. TSL is expected to be formed from twinning planes of long-range order, which leads to the formation of series homojunctions with short spacing. In this case, both excited electrons and holes can be efficiently separated in shorter travelling distance before they undergo recombination. Such densely distributed homojunctions are obviously advantageous than the single buried-in homojunction as reported by Lin et al . [52] , which introduced a thin p-type layer on n-type α-Fe 2 O 3 and created a built-in field. In conclusion, we demonstrated the efficient charge separation and therefore very high hydrogen production without noble metal loading over our twinning Cd 0.5 Zn 0.5 S nanorod photocatalysts. The key to this achievement is the successful formation of high-density (111)/[11-2]-type TSL in certain dimension. Long-range ordered twinning planes with preferred [111] orientation leads to near periodical and dense distribution of a series of homojunctions. These homojunctions have been demonstrated to be very efficient in separating photo-generated charges and contributed to prolonged lifetime of both photo-generated electrons and holes. It is predicted that even higher photocatalytic activity could be achieved if larger aspect ratios, that is, longer Cd 0.5 Zn 0.5 S twinned nanorods, could be obtained. The ability to form such a homojunction by twin planes in a semiconductor presents a promising strategy for precise band engineering without introducing foreign materials or elements as required by traditional heterojunctions and provides new insight into the fabrication of novel structures for photocatalytic and photoelectrochemical applications. Syntheses Cd 0.5 Zn 0.5 S-EN10 nanocrystals were prepared by sequentially adding 10 ml of EN and 25 mmol thioacetamide of to a 40-ml aqueous solution containing 10 mmol of cadmium acetate (Cd(CH 3 COO) 2 ) and 10 mmol of zinc acetate (Zn(CH 3 COO) 2 ). The total volume of the reaction was adjusted to be 60 ml by introducing additional water. The entire process was carried out under magnetic stirring. The reaction mixture was further stirred for 20 min, sealed in a 100 ml-capacity Teflon-lined autoclave, and heated to 230 °C at a ramping speed of 30 °C min −1 in the presence of microwave irradiation. The reaction was allowed to proceed for 30 min. After cooling, the product was separated by centrifugation, washed several times with deionized water and ethanol, and dried at 80 °C for 5 h in a vacuum oven. Preparation of other Cd 1− x Zn x S-EN10 nanocrystals is the same with the synthesis of Cd 0.5 Zn 0.5 S-EN10 nanocrystal except employing a different molar ratio of Cd(CH 3 COO) 2 /Zn(CH 3 COO) 2 . For the synthesis of other Cd 0.5 Zn 0.5 S photocatalysts for comparison, the processes were similar to that of Cd 0.5 Zn 0.5 S-EN10 synthesis, except that 5 and 20 ml of EN, and 10 ml of sodium hydroxide (NaOH, 4 M) were used (instead of 10 ml EN). The total volume of the reaction was also adjusted to be 60 ml by introducing additional water. Photocatalytic reactions Photocatalytic reactions of hydrogen production from water were conducted in a gas-closed system with a side irradiation Pyrex cell (using PLS-SXE300/300UV Xe lamp irradiation) at 35 °C. The photocatalyst powder (0.1 g) was dispersed with a magnetic stirrer in an aqueous solution (180 ml) containing sodium sulphide (Na 2 S, 0.35 M) and sodium sulphite (Na 2 SO 3 , 0.25 M) as electron donors. The photocatalysts were irradiated with visible light ( λ ≥430 nm) through a cutoff filter from the Xe lamp. The intensity and number of photons of the two light sources were measured with a fiber optic spectrometer. The amount of H 2 gas was determined by online thermal conductivity detector gas chromatography (NaX zeolite column, thermal conductivity detector detector, and N 2 carrier) or drainage. QEs were measured using 425 nm band pass filters and an irradiation meter and were defined by equation (1): where N H is the number of evolved H 2 molecules and N P is the number of incident photons. No H 2 evolution was detected under blank experiments carried out in the absence of catalysts or /and visible light irradiation. The catalytic feature of Cd 0.5 Zn 0.5 S twinning rods was further certified by their unchanged structural, optical and morphologic properties, recovered and characterized after 20-h hydrogen production (see Supplementary Fig. S9 ). Modelling details The rotational twin boundary was modelled by a 12H supercell, as shown in Fig. 5a and Supplementary Fig. S3 . Two equivalent boundaries were actually included in the supercell with each boundary well separated. Charge densities at the VBM and CBM and a potential barrier across the twin boundary were calculated using the Vienna ab initio simulation package [53] , [54] . Generalized gradient approximation [55] within density functional theory and the projector augmented wave potentials [56] were used [55] , [56] . A kinetic energy cutoff of 380 eV was chosen, and a 9 × 9 × 1 Monkhorst–Park k-point mesh was used to sample the hexagonal two-dimensional Brillouin zone [57] . The twin boundary was fully relaxed until the force acting on ions was smaller than 0.01 eV Å −1 . The band decomposed charge density was extracted to depict charge distribution along the direction normal to the boundary. The macro-averaged total potential was used to determine the potential barrier across the boundary. The ZB/WZ interface was modeled by a (3C) 2 (2H) 3 supercell. The band offset across the ZB/WZ interface was obtained using macro-averaged total potential by combining the interface and individual ZB and WZ bulk calculations [58] . Characterizations The X-ray diffraction patterns of the prepared photocatalysts were confirmed by an X’Pert PRO diffractometer using Cu Ka (λ=0.1538, nm) radiation with a constant instrument parameter. All samples were scanned between 10° and 90° with a step size of 0.033°. Diffuse reflectance ultraviolet-vis spectra were obtained on a Hitachi U-4100 spectrometer equipped with a laboratory-sphere diffuse reflectance accessory. The crystallite morphologic micrographs were observed by JEOL JSM-6700F field emission SEM). TEM JEM-3010 and transmission electron microscope FEI Tecnai F30. STEM and EDX analyses were performed using an ARM200 microscope with a STEM Cs corrector (JEOL, Tokyo, Japan). The room temperature photoluminescent emission spectra and time-resolved photoluminescent emission decay spectra were measured on a PTI QM-4 fluorescence spectrophotometer. How to cite this article: Liu, M. et al . Twin-induced one-dimensional homojunctions yield high quantum efficiency for solar hydrogen generation. Nat. Commun. 4:2278 doi: 10.1038/ncomms3278 (2013).